Identification of genetic variants associated with alternative splicing using sQTLseekeR Identification of genetic variants affecting splicing in RNA sequencing population studies is still in its infancy. Splicing phenotype is more complex than gene expression and ought to be treated as a multivariate phenotype to be recapitulated completely. Here we represent the splicing pattern of a gene as the distribution of the relative abundances of a gene’s alternative transcript isoforms. We develop a statistical framework that uses a distance-based approach to compute the variability of splicing ratios across observations, and a non-parametric analogue to multivariate analysis of variance. We implement this approach in the R package sQTLseekeR and use it to analyze RNA-Seq data from the Geuvadis project in 465 individuals. We identify hundreds of single nucleotide polymorphisms (SNPs) as splicing QTLs (sQTLs), including some falling in genome-wide association study SNPs. By developing the appropriate metrics, we show that sQTLseekeR compares favorably with existing methods that rely on univariate approaches, predicting variants that behave as expected from mutations affecting splicing. RNA-Seq has increased the resolution at which transcriptomes can be monitored, providing quantification of the abundances of individual splicing events (splice junctions, exons, transcripts, and so on), in addition to global gene expression levels. If transcriptomes are monitored in large cohorts of genotyped individuals, methods can be employed to identify genetic variants affecting the splicing pattern of genes. Splicing alterations may have a phenotypic impact, even in the absence of changes in overall gene expression. Indeed, splicing defects caused by DNA mutations are at the root of many Mendelian disorders [1] , [2] , such as cystic fibrosis [3] or progeria [4] . Thus, eQTL methods have been recently employed to identify single nucleotide polymorphism (SNPs) that are associated to changes in the inclusion levels of exons [5] , [6] . Exons, however, are not independent transcriptional units, but they are linked into transcripts. Dramatic changes may occur, therefore, in the splicing pattern of a gene that are not reflected in changes in the inclusion levels of individual exons ( Fig. 1 ). To overcome this limitation, eQTL methods have also been employed to test association between SNPs and abundances of individual transcript isoforms [7] , [8] , [9] . To control for the effect of overall gene expression, the phenotype actually tested is the ratio of the transcript isoform’s abundance over total gene expression. Testing independently, each transcript isoform ignores, however, the strongly correlated structure of the relative abundances of splicing isoforms. This is likely to lead to loss of power to detect QTLs related to splicing.The effect may be particularly important in genes with a large number of splice isoforms (most human genes) in which subtle splicing changes are distributed among many of them. 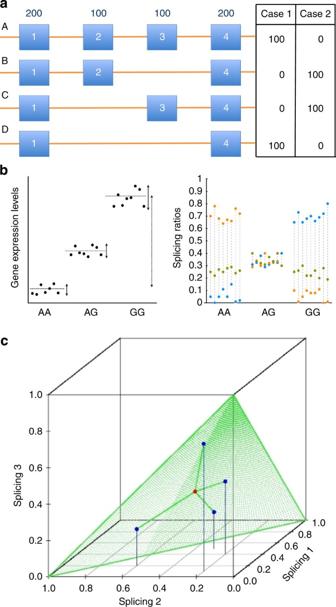Figure 1: sQTLs and the sQTLseekeR approach. (a) Alternative transcript versus alternative exon usage. A gene with four isoforms (A,B,C and D), whose abundances is measured in two different individuals. In individual 1, only isoforms A and D are found with abundance 100 (say copies per cell) each. In individual 2, only isoforms B and C are found, also with abundance 100 each. The splicing pattern in the two individuals is completely different. However, exons abundances (on top of the exon, in the figure) are identical in the two individuals. (b) Testing the association between the distribution of the relative abundances of a gene’s transcript isoforms and a SNP. Left panel. The expression level of gene (yaxis) measured on individuals polymorphic at a given genomic site (SNP,xaxis). There is a clear association between genotype and expression. To test for association between the SNP and gene expression, the variance of the expression within the genotypes (solid arrows) and between the genotypes (dashed arrow) can be compared. Right panel. The abundances of each individual transcript isoform (blue, green and orange) for a gene measured in individuals polymorphic at a genomic site (xaxis). The relative abundances of each transcript (splicing ratios) are computed relative to the total abundance of the gene (yaxis). There is a clear association between genotypes and splicing ratios. The AA genotypes express predominantly the orange isoform, while the GG genotypes express predominantly the blue isoform. The heterozygous express the two isoforms at similar levels, and similar to the levels of the green isoform—whose relative abundance does not appear to be affected by the genotype. In our approach, association between SNP and splicing ratios is also tested by comparing within and between genotype variabilities of the splicing ratios. See Methods. (c) The space of the splicing ratios of a gene with three isoforms. Four samples/observations (blue points) are represented. The point in red is the centroid of the samples and the green triangle represents the 2-simplex space. The sum of squared distances (SS) between the observations and the centroid is the basic measure of variability used in our approach. Figure 1: sQTLs and the sQTLseekeR approach. ( a ) Alternative transcript versus alternative exon usage. A gene with four isoforms (A,B,C and D), whose abundances is measured in two different individuals. In individual 1, only isoforms A and D are found with abundance 100 (say copies per cell) each. In individual 2, only isoforms B and C are found, also with abundance 100 each. The splicing pattern in the two individuals is completely different. However, exons abundances (on top of the exon, in the figure) are identical in the two individuals. ( b ) Testing the association between the distribution of the relative abundances of a gene’s transcript isoforms and a SNP. Left panel. The expression level of gene ( y axis) measured on individuals polymorphic at a given genomic site (SNP, x axis). There is a clear association between genotype and expression. To test for association between the SNP and gene expression, the variance of the expression within the genotypes (solid arrows) and between the genotypes (dashed arrow) can be compared. Right panel. The abundances of each individual transcript isoform (blue, green and orange) for a gene measured in individuals polymorphic at a genomic site ( x axis). The relative abundances of each transcript (splicing ratios) are computed relative to the total abundance of the gene ( y axis). There is a clear association between genotypes and splicing ratios. The AA genotypes express predominantly the orange isoform, while the GG genotypes express predominantly the blue isoform. The heterozygous express the two isoforms at similar levels, and similar to the levels of the green isoform—whose relative abundance does not appear to be affected by the genotype. In our approach, association between SNP and splicing ratios is also tested by comparing within and between genotype variabilities of the splicing ratios. See Methods. ( c ) The space of the splicing ratios of a gene with three isoforms. Four samples/observations (blue points) are represented. The point in red is the centroid of the samples and the green triangle represents the 2-simplex space. The sum of squared distances ( SS ) between the observations and the centroid is the basic measure of variability used in our approach. Full size image Here, to fully capture splicing variation, we use the distribution of the relative abundances of the gene’s splicing isoforms (to which we refer here as ‘splicing ratios’, Fig. 1 ) as the splicing phenotype. Most other quantitative splicing-related phenotypes (exon inclusion, usage of alternative splice forms, abundances of individual transcript isoforms, and so on) can be derived from it (and from the overall expression of the gene). Then, we address the problem of identifying splicing-related QTLs as the problem of identifying genetic variants that are associated to changes in the splicing ratios of genes ( Fig. 1 ). We will refer to these variants, as splicing QTLs (sQTLs). Because these ratios configure a multivariate phenotype, classical eQTL methods cannot be employed. We develop an alternative framework, which includes two main components. First, we define the variability of splicing ratios of a gene along a number of observations using a distance-based approach originally introduced by Anderson [10] , [11] to test for the differences in the relative abundance of organisms across ecological samples (see also Gonzalez-Porta [12] ). Second, to test for the association between a SNP and a gene, we compare the variability of the splicing ratios within genotypes with the variability between genotype using a non-parametric analogue to the analysis of the variance [10] . Based on this theoretical framework, we implement sQTLseekeR, an R package to identify sQTLs in transcriptome population studies. It can be downloaded from http://big.crg.cat/computational_biology_of_rna_processing/sqtlseeker . We use this approach in a panel of 465 lymphoblastoid cell lines samples from five populations of the 1,000 Genomes Project [13] , whose transcriptome has been recently monitored by RNA-Seq in the framework of the Geuvadis Project [8] . The results obtained demonstrate the power of our approach. SNPs within a tested gene are about 100-fold more likely to be sQTLs for that gene that SNPs mapping to another gene consistent with the assumption that SNPs affecting the splicing of a gene will most likely fall within the gene’s primary transcript sequence. Moreover, the sQTLs that we identify as significant are more exonic or closer to exonic boundaries, alter splicing in the expected direction when occurring within splice sites and are highly enriched for genome-wide association study (GWAS) SNPs compared with non (significant) sQTLs. Benchmarks using the Geuvadis data, as well as simulations, show that sQTLseekeR outperforms other existing methods based on an univariate approach. sQTLs and sQTLseekeR Let’s assume a gene with n transcript isoforms, and let x ij the abundance of the transcript i (that is, the number of copies) in a given individual (condition, sample, observation...) j , the relative abundance of transcript i in individual j is . We will refer to the relative transcript abundances f 1 j ,···, f nj as the gene splicing ratios. Obviously, for any individual j . We define here a splicing QTL (sQTL) as a SNP that associates with changes in the splicing ratios of a target gene ( Fig. 1 ). As in many eQTL method, we assess SNP–gene pairs for sQTLs by comparing the variance of the splicing ratios within genotypes with the variance between genotypes. The problem is that, in contrast to gene expression values, splicing ratios are not scalar, but vectors. Thus, to compute the variability of splicing ratios across observation, we follow here a distance-based approach introduced by Anderson [10] , and that we have recently adapted to investigate variability of splicing in human populations [12] . Given the splicing ratios of a gene in a number of individuals, we represent each individual as a point in a multidimensional space, whose coordinates are the ratios of each splicing isoform in the target gene. The variability in the splicing ratios of the gene across the individuals is the mean of the squared distances of the individual splicing ratios to the centroid of all individuals ( Fig. 1 ). As a dissimilarity measure, we use the Hellinger distance, which defines the underlying metric of our approach (see Methods). To assess the association between the genotype at a given SNP, and the splicing ratios of a given gene, we use the Anderson test for location comparison [10] . The test is similar to a multivariate analysis of variance (MANOVA) without assuming any probabilistic distribution for the splicing ratios: a pseudo-F ratio score measures the relative difference between the within-group variability and the between-group variability. The between-group variability corresponds to the mean of the squared distances of the within-group centroids to the global centroid. This factorial model with the genotypes as levels of the factor appears more appropriate than a regression model with the genotypes as independent variables because, in contrast to gene expression values, splicing ratios do not strictly follow the additive model. Given the nature of our data, multivariate vectors of proportions, a non-parametric approach appears superior to a classical MANOVA. Indeed, we compared the synthetic null distributions of the classical MANOVA on the real splicing ratios after shuffling the genotype groups, with simulated null distributions using data generated under a Gaussian model, and found the two distributions to be vastly divergent (Methods). Since the Anderson location test is sensitive to heterogeneity in the dispersion of the points, we use a test of homogeneity also developed by Anderson [14] . Thus, we compute and adjust independently the location and homogeneity tests. While the significance of the pseudo-F score is typically assessed using a permutation procedure, we have here implemented an asymptotic approximation [14] that speeds up the test computation 80-fold, while producing nearly identical results (Methods). Based on this theoretical framework, we have implemented sQTLseekeR, an R package to identify sQTLs in transcriptome population studies. For each gene–SNP pair, sQTLseekeR computes the pseudo-F score described above and assesses its significance. After all gene–SNP pairs considered are tested, the P values for all genes and all SNPs are pooled together and controlled for false discovery rate (FDR). Significant sQTLs are reported (see Methods for details). sQTLs by sQTLseekeR in the 1000 genomes project We used sQTLseekeR to analyze 465 lymphoblastoid cell lines samples that originated from individuals from five populations of the 1000 Genomes Project [13] ( Table 1 ), whose transcriptome has been recently monitored by RNA-Seq in the framework of the Geuvadis Project [8] . We ran sQTLseekeR on the SNPs and transcript quantifications produced by this project. Under the assumption that SNPs that directly affect splicing are likely to be carried out to the sequence of the primary transcript, we tested only SNPs within the body of the gene (exons and introns) plus 5,000 bp upstream from the transcription start site (TSS) and 5,000 bp downstream from the transcription termination site. Furthermore, we considered only genes with at least two alternative splicing (AS) isoforms and exhibiting a minimum splicing variability across individuals, as well as only bi-allelic SNPs creating at least two genotypes, each of which present in at least five individuals. Table 1 sQTLs in Geuvadis populations. Full size table sQTLseekeR was run separately in each population. On average, about 1.3 M SNPs, 10,012 genes and 140 SNPs per gene were tested in each population ( Table 1 and Supplementary Table 1 ). It took on average 4 h to analyze each population, using 16 cores (2 Gb 2.70 GHz nodes). We found on average 2,900 and 1,950 significant associations across populations at a FDR of 5 and 1%, respectively. Some examples of sQTLs are displayed in Fig. 2 . We found high recurrence of sQTLs across the five investigated populations. Using the π 1 estimate [15] , we found averages of 92% sQTL sharing between European populations and of 85% between Yoruban and European populations ( Fig. 3 ). We also observed more European-specific than African-specific sQTLs. sQTLseekeR can detect SNPs affecting the entire transcript structure, including alternative TSS or transcription termination sites. We have used the AStalavista software [16] , to characterize the types of alternative transcript events detected by sQTLseekeR (Methods). We have found that about 66% of sQTLs involve only changes in alternative first or last exon usage, or in untranslated regions (UTRs). Among the remaining 34% corresponding to splicing of internal exons, the majority involve complex events but some simple events are also detected, for example, 13% of sQTLs are associated to exon skipping ( Fig. 4 ). Note that sQTLs can be associated to more than one event within the transcripts (Methods). For instance, a variant could affect the splicing of an exon as well as the length of the 3′ UTR. On average, we found sQTLs to be associated to 1.7 events. As a control, we randomly selected pairs of transcripts from the genes hosting detected sQTLs, and compared them using the same approach. We found that sQTLs involve more splicing-related events than expected by chance (34% compared with 20%) and that they tend to be associated to a larger number of events than expected by chance (1.7 compared with 1.1). The proportion of sQTLs associated to each type of event is shown in Fig. 4 . 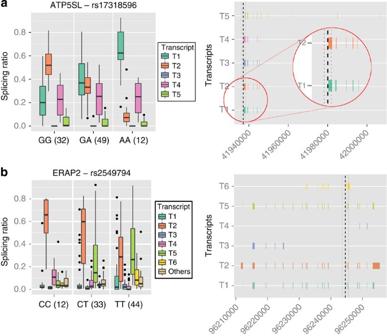Figure 2: sQTL examples. In the left panels, we represent as box-plots the distribution of the splicing ratios of the candidate gene in a selected population. The distributions are given separately for each genotype and the number of tested individuals in each genotype is given in parenthesis next to the genotype. Each splicing isoform is represented by a different color. When there are more than six transcripts, the lowly expressed ones are merged into a single one for clarity sake. The right panels show the exonic structure of the transcripts along with the location of the sQTL SNP (dotted line). (a) Association between the SNPrs17318596, and theATP5S-like gene. In the left panel we represent as box-plots the distribution of the splicing ratios of this gene in the GBR population. The distributions are given separately for each genotype and the number of tested individuals in each genotype is given in parenthesis next to the genotype. Each splicing isoform is represented by a different color. The SNPrs17318596has been found associated with height37, but no association with gene expression has been reported for it. We have detected, however, in the GBR and TSI populations, a strong effect of the SNP in relative abundance of the transcripts in this gene. The isoform T1 (green) is the dominant one in the individuals with the AA genotype, it captures on average 62% of the total expression of the gene while it captures only about 20% in the individuals with the GG genotype. Conversely, the isoform T2 (orange) captures more than 50% of the expression in the GG genotype but only about 5% in the AA genotype.The right panel shows the exonic structure of the transcripts along with the location of the sQTL SNP (dotted line). The isoform T2 skips the third exon compared with the isoform T1. (b) Theendoplasmic reticulum aminopeptidase 2gene, already known to host sQTLs17. We detected the SNPrs2549794, known to be associated to Crohn disease37, as a sQTL in CEU, FIN, TSI and YRI (displayed in the box-plot) populations. Figure 2: sQTL examples. In the left panels, we represent as box-plots the distribution of the splicing ratios of the candidate gene in a selected population. The distributions are given separately for each genotype and the number of tested individuals in each genotype is given in parenthesis next to the genotype. Each splicing isoform is represented by a different color. When there are more than six transcripts, the lowly expressed ones are merged into a single one for clarity sake. The right panels show the exonic structure of the transcripts along with the location of the sQTL SNP (dotted line). ( a ) Association between the SNP rs17318596 , and the ATP5S- like gene. In the left panel we represent as box-plots the distribution of the splicing ratios of this gene in the GBR population. The distributions are given separately for each genotype and the number of tested individuals in each genotype is given in parenthesis next to the genotype. Each splicing isoform is represented by a different color. The SNP rs17318596 has been found associated with height [37] , but no association with gene expression has been reported for it. We have detected, however, in the GBR and TSI populations, a strong effect of the SNP in relative abundance of the transcripts in this gene. The isoform T1 (green) is the dominant one in the individuals with the AA genotype, it captures on average 62% of the total expression of the gene while it captures only about 20% in the individuals with the GG genotype. Conversely, the isoform T2 (orange) captures more than 50% of the expression in the GG genotype but only about 5% in the AA genotype.The right panel shows the exonic structure of the transcripts along with the location of the sQTL SNP (dotted line). The isoform T2 skips the third exon compared with the isoform T1. ( b ) The endoplasmic reticulum aminopeptidase 2 gene, already known to host sQTLs [17] . We detected the SNP rs2549794 , known to be associated to Crohn disease [37] , as a sQTL in CEU, FIN, TSI and YRI (displayed in the box-plot) populations. 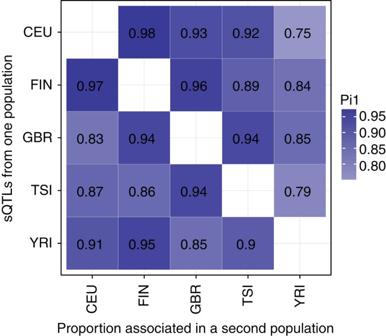Figure 3: sQTL sharing between populations. Proportion of true associations in one population among the significant associations (FDR 5%) in another population. Full size image Figure 3: sQTL sharing between populations. Proportion of true associations in one population among the significant associations (FDR 5%) in another population. 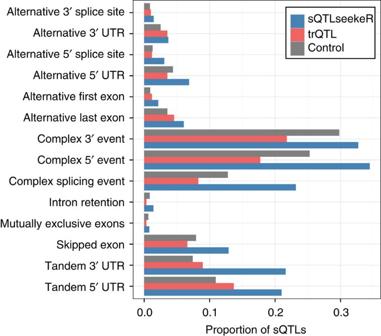Figure 4: Classification of the major transcript changes. A same sQTL can be associated to several distinct events, hence can be counted in different categories. On thexaxis, the proportion of sQTLs associated to each type of major AS event (yaxis) at a FDR of 5%. The control track was computed choosing randomly two transcripts among the expressed ones for genes hosting a sQTL. We note that the bars are consistently higher for sQTLseeker, meaning that a sQTL is more likely associated with several major AS events compared with trQTL or random distribution. A description of each event is shown inSupplementary Fig. 5. Full size image Figure 4: Classification of the major transcript changes. A same sQTL can be associated to several distinct events, hence can be counted in different categories. On the x axis, the proportion of sQTLs associated to each type of major AS event ( y axis) at a FDR of 5%. The control track was computed choosing randomly two transcripts among the expressed ones for genes hosting a sQTL. We note that the bars are consistently higher for sQTLseeker, meaning that a sQTL is more likely associated with several major AS events compared with trQTL or random distribution. A description of each event is shown in Supplementary Fig. 5 . Full size image A number of metrics support the quality of the sQTLs discovered by sQTLseekeR ( Table 2 ). First and consistent with the biological assumption that SNPs affecting splicing are likely to be mostly in cis , we found on average 100-fold more sQTLs when testing SNPs within the same gene, than when we tested SNPs occurring in a different gene ( Table 1 ). A functional analysis of the genes hosting these apparently false positive ‘trans sQTLs’ showed that around one fourth (25/107) are involved in RNA transcription and processing ( Supplementary Table 2 ), suggesting that a fraction of these ‘trans’ mutations could indeed affect the splicing of the tested gene. Second, we found sQTLs to be significantly more exonic, closer to exonic boundaries and to overlap splice sites more often that non sQTL SNPs ( Table 2 and Fig. 5 ). Third, we observed that the absolute change in the strength of splice sites induced by SNPs was significantly higher in sQTLs than in non-sQTLs, and more strikingly, that SNPs increasing (decreasing) the strength of the splice site, also increase (decrease) its relative usage, specifically when they are sQTLs ( Table 2 ). Fourth, we found 11% of all sQTLs within 1 Kb of GWAS SNPs-a striking 24-fold enrichement of the proportion found for non-sQTL SNPs. Finally, we compared our sQTLs with the sQTLs found by Kwan et al [17] in Hapmap samples, the transcriptomes of which were monitored by exon arrays. Thirteen13 SNPs from the validated set in this study were also tested by us: nine of them (70%) reached nominal significance ( P value<0.05). Considering that the monitoring technology (expression and genotypes), methodology and samples are different, the overlap is substantial. For comparison, monitoring exactly the same phenotype, the same set of samples and using the same statistical method, Pickrell et al. [6] were able to replicate with RNA-Seq, 70% of eQTLs obtained from microarrays. Table 2 Enrichment in splicing-related features in sQTLs identified by sQTLseeker in Geuvadis, and Geuvadis trQTLs. 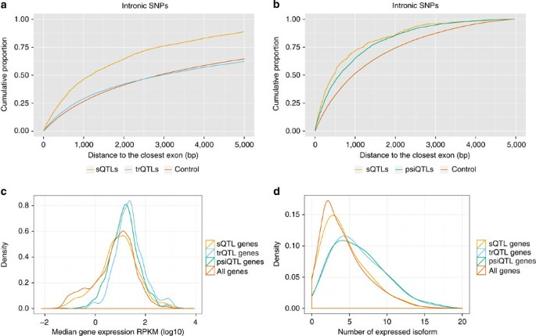Figure 5: Location and expression profile of sQTLs. (a) Distance to exons of intronic sQTLs and trQTLs. Cumulative proportion of intronic sQTLs and trQTLs at 5% FDR that are at a given distance of the closest exon. The control SNPs were non-QTL intronic SNPs with matched minor allele frequencies. (b) Distance to exons of intronic sQTLs and psiQTLs. Cumulative proportion of intronic sQTLs and psiQTLs at 1% FDR that are at a given distance of the closest exon. Only SNPs tested by both methods are compared (about 12% of the total SNPs tested by sQTLseekeR). (c) Distribution of gene expression for genes hosting sQTLs, trQTLs and psiQTLs, compared with all genes. (d) Distribution of the number of expressed isoforms for genes hosting sQTLs, trQTLs and psiQTLs, compared with all genes. Isoforms are considered expressed if their RPKM >0.01. Full size table Figure 5: Location and expression profile of sQTLs. ( a ) Distance to exons of intronic sQTLs and trQTLs. Cumulative proportion of intronic sQTLs and trQTLs at 5% FDR that are at a given distance of the closest exon. The control SNPs were non-QTL intronic SNPs with matched minor allele frequencies. ( b ) Distance to exons of intronic sQTLs and psiQTLs. Cumulative proportion of intronic sQTLs and psiQTLs at 1% FDR that are at a given distance of the closest exon. Only SNPs tested by both methods are compared (about 12% of the total SNPs tested by sQTLseekeR). ( c ) Distribution of gene expression for genes hosting sQTLs, trQTLs and psiQTLs, compared with all genes. (d) Distribution of the number of expressed isoforms for genes hosting sQTLs, trQTLs and psiQTLs, compared with all genes. Isoforms are considered expressed if their RPKM >0.01. Full size image Benchmarks of sQTLseekeR There are no comparable methods to detect genetic variants associated to changes in splicing ratios. We have, however, compared the sQTLs found using sQTLseekeR with the transcript ratio QTLs (trQTLs) obtained in the Geuvadis project [8] . In Geuvadis, each transcript isoform is tested independently in a univariate framework—an approach that has also been recently employed in Battle et al [9] . While this approach has led to the discovery of relevant association, we found our sQTLs to exhibit somehow superior enrichment for nearly all splicing-related features ( Table 2 and Fig. 5 ). To further compare the univariate approaches, as in the in the Geuvadis project [8] and Battle et al. [9] , with our multivariate approach we have used simulations. We have considered genes with different numbers of isoforms (3,4,7,10 and 15) and compared the capacity of the two approaches to detect significant changes (associations) in the relative frequencies of the isoforms when comparing two simulated populations of 40 individuals each. The causistic is almost unlimited but, we have simulated four main scenarios, which we believe describe realistic patterns of changes in splicing ratios, and explored them exhaustively by varying the magnitude of the effect. In total, we have simulated 400 configurations, each configuration simulated 500 times. See sec:methods for details. The multivariate approach consistently detects more significant associations in nearly all configurations than the univariate approach. For some effect sizes, the univariate approach misses almost half of the associations identified by the multivariate approach ( Fig. 6 ). At these effect sizes, biologically relevant associations are likely to exist (see Methods and Supplementary Fig. 1 ). 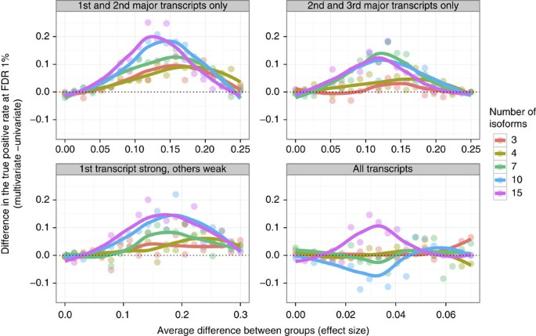Figure 6: Detected associations by simulated univariate (as in trQTLs) and multivariate (as in sQTLs) approaches. Gain in the proportion of detected association (yaxis) when using multivariate approach versus univariate approach. We simulated two populations for genes expressing 3, 4, 7 or 10 transcripts (columns) when the transcript ratios are shifted by a certain value (effect size,xaxis) from one population to the other following four different scenarios (rows): ‘all transcripts’: the splicing ratios of all transcripts change with the same intensity in the second population compared with the first. ‘first and second major transcripts only’: only the splicing ratios of the first two major transcripts, are shifted in the second population. ‘second and third major transcripts only’: only the splicing ratios of the second and third major isoforms are changed in the second population. ‘first transcript strong, others weak’: the splicing ratios of all transcripts are shifted but the value of the change in the major isoform is distributed equally among the rest of the isoforms, that is, the major transcript changes strongly while the other transcripts change slightly. For each configuration, 500 genes with different splicing ratios were pooled with 4,500 non-associated genes. After multiple testing correction, we compute the true positive rate (that is, proportion of true association detected) using a FDR threshold of 1%. The plot displays the difference between multivariate TPR and univariate TPR. (Positive values correspond to higher TPR in the multivariate approach). The curves are obtained using a LOESS model. Figure 6: Detected associations by simulated univariate (as in trQTLs) and multivariate (as in sQTLs) approaches. Gain in the proportion of detected association ( y axis) when using multivariate approach versus univariate approach. We simulated two populations for genes expressing 3, 4, 7 or 10 transcripts (columns) when the transcript ratios are shifted by a certain value (effect size, x axis) from one population to the other following four different scenarios (rows): ‘all transcripts’: the splicing ratios of all transcripts change with the same intensity in the second population compared with the first. ‘first and second major transcripts only’: only the splicing ratios of the first two major transcripts, are shifted in the second population. ‘second and third major transcripts only’: only the splicing ratios of the second and third major isoforms are changed in the second population. ‘first transcript strong, others weak’: the splicing ratios of all transcripts are shifted but the value of the change in the major isoform is distributed equally among the rest of the isoforms, that is, the major transcript changes strongly while the other transcripts change slightly. For each configuration, 500 genes with different splicing ratios were pooled with 4,500 non-associated genes. After multiple testing correction, we compute the true positive rate (that is, proportion of true association detected) using a FDR threshold of 1%. The plot displays the difference between multivariate TPR and univariate TPR. (Positive values correspond to higher TPR in the multivariate approach). The curves are obtained using a LOESS model. Full size image We have also compared our method with an exon-based method, related to that employed in Pickrell et al [6] . We have specifically implemented an approach recently described in Zhao et al . [5] and computed exon QTLs when measuring inclusion using the percent spliced in measure (psiQTLs) on Geuvadis populations. A direct comparison is more difficult here because different sets of gene/SNPs are tested by each method (see Methods and Table 3 ). Thus, the overlap between psiQTLs and sQTLs is only moderate, which emphasizes the complementarity of the two approaches. However, when considering only the SNPs tested by the two methods (about 12% of all those tested by sQTLseekeR), sQTLs exhibit also superior enrichment for nearly all splicing-related features compared with psiQTLs ( Table 4 and Fig. 5 ). We finally investigated the effect of gene expression and number of expressed isoforms. We found that sQTLseekeR can detect sQTLs along the entire range of gene expression and number of isoforms. In contrast, trQTLs and psiQTLs appear to require higher levels of gene expression and larger numbers of isoforms to be detected ( Fig. 5 ). Table 3 psiQTLs in Geuvadis populations. Full size table Table 4 Enrichment in splicing-related features in sQTLs compared with psiQTLs in Geuvadis. Full size table By construction, psiQTLs correspond almost exclusively to exon-skipping events. In contrast, trQTLs, can correspond in principle, to any type of alternative splice event. We have categorized trQTLs as described above. Compared with sQTLs by sQTLseekeR, only 16% of trQTLs correspond to internal splicing events (compared with 34% for sQTLs), and on average trQTLs are associated to 1.1 alternative transcript even (compared with 1.7 for sQTLs, see Fig. 4 ). These results indicate that sQTLseekeR is able to detect sQTLs associated with complex splicing events that escape exon centric and/or univariate approaches. We have developed a statistical framework for identifying genetic variants that are associated to changes in the relative abundances of the AS isoforms (what we call sQTLs). We have shown that this approach, which captures the intrinsic multivariate nature of the splicing phenotype, compares favorably with existing exon- and transcript-based methods that employ an univariate approach. Deriving abundances of transcript isoforms from RNA-Seq is, however, a difficult problem [18] , and it is indeed unclear how reliable available methods are [19] . Transcript quantifications, are likely to be, in any case, less robust and noisier than direct measurements of exon inclusion levels. This could indeed result in decreased power to detect associations. Therefore, we currently see sQTLseekeR as a complement to other existing methods, and our results do show that it is able to detect associations that are invisible to univariate exon centric approaches. Using sQTLseekeR, we identified hundreds of sQTLs, some of which falling in GWAS SNPs that have not been previously predicted to be eQTLs. This underlines that the phenotypic impact of many biologically and even medically relevant mutations is not necessarily mediated by alternations in the overall gene expression, but by a shift in the balance of the relative abundances of the gene’s alternative transcript isoforms. While we believe that we approach for the first time the particular case of multivariate molecular phenotypes as such, the problem of detecting genetic association with multivariate phenotypes has received previous attention. For instance, mixed effect models [20] , generalized estimating equations [21] or combinations of univariate association tests [22] have been used when the multivariate trait of interest is a collection of single numeric or/and qualitative measures. More recently, multivariate methods have been developed within the eQTL field. Thus Chun and Keles [23] apply a multivariate method to reduce the dimension of an eQTL problem by clustering genes with similar expression patterns, and therefore reduce the number of tests that need to be performed. Multivariate methods have also been developed to address the multiple tissue eQTL problem [24] , [25] , [26] . While, in principle, it is theoretically possible to re-engineer some of these methods in a splicing QTL framework, a number of features in the sQTL problem make our approach more appropriate. First, the splicing ratios are correlated within every gene, while the ratios of different genes may be correlated only in some cases. These different levels of dependence make it difficult to define a general model to analyze jointly all the genes. Second, the multivariate dimension of the phenotypes (the number of alternative transcript isoforms) is different from one gene to the other, which makes difficult the fitting of a common model if the genes are analyzed separately. Third, the splicing ratios are complex variables unlikely to fit normality. In contrast, the Anderson’s approach followed by the multiple testing adjustment provides the desired homogeneous assessment of associations, while retaining the conceptual simplicity of an ANOVA analysis. We have explicitly opted for developing a splicing QTL tool, which is independent from the underlying program used to obtain transcript quantifications from RNA-Seq reads. There are quantification programs, however, which incorporate specialized methods to identify differentially expressed isoforms between samples, such as MISO [27] and CuffDiff [28] . They could, in principle, be engineered in a sQTL framework. However, they suffer from the limitation that they are limited to the comparison of two groups and designed for small sample sizes (a few replicates per group), while in QTL analysis most tests include three genotype groups and large sample sizes. The Anderson test that we use in our approach, in contrast, is able to handle much more complex factorial designs, including comparisons between multiple groups. It is also designed to integrate a large number of samples. Being model free, it can be used with any transcript quantification program, including MISO and Cufflinks. Actually, we believe that the framework developed here is general enough to be employed as an appropriate alternative to analyze in general multivariate phenotypes when the components of the trait are relative proportions. For instance, the expression of a given gene in different tissues or across different time points could be considered a multivariate phenotype and converted to proportions when normalized to the sum of expressions. Our approach could be directly employed for joint analysis of gene expression across tissues, as an alternative to the methods by Ackermann et al. [24] and Sul et al. [26] In a more complex scenario, it could also be used to identify SNPs affecting expression networks, where the multivariate phenotype is the relative expression of gene compared with the total expression output of the network. Within our framework, it should be possible to robustly compare networks of different size and made of different genes. sQTLseekeR could also be used to identify host SNPs that affect the population structure of a metagenomic community, which is usually described as the relative abundances of microbial species. In metatranscriptome studies, it could be used to assess association with the cumulative expression of families of orthologous genes across the community. Beyond molecular phenotypes, the method could also be used to identify pleiotropic SNPs or SNPs influencing ‘allometric traits’. For instance, the primary skeletal components of height in humans are the long bones of the leg, the vertebral column and the skull. The length of each of these components, in turn, results from the contribution of other most basic traits. The relative contribution to each of these traits to total height conforms a multivariate phenotype analogous to splicing ratios. Genetic variants influencing the relative scaling between these components [29] could thus be identified using the method delineated here. Anomalous scaling (for instance between vertebral and invertebral disk height) could result in pathological conditions [30] . The initial implementation of sQTLseekeR can obviously be further enhanced. Currently, the method does not take into account the confidence of transcript quantifications—which often depends on the sequence coverage. The Hellinger distance has ‘a priori’ good properties in the case of the splicing ratios, but other distances could be evaluated in the context of sQTL discovery. We could also explore methods alternatives to Storey’s qvalue [31] for FDR correction, such as Efron’s FDR. While we have used here a one-way factorial model, in which each population is tested separately, Anderson’s location test allows for higher order factorial models. For instance, we could have implemented a two-way model, with the population as a second factor. Testing the pooled populations appears as a more natural approach to identify population specific sQTLs, benefiting from a greater samples size, and thus increased power. As multivariate distributions of relative frequencies may be particularly appropriate to describe phenotypic relationships at many different levels, from molecular to organismic, many avenues of research remain open to develop efficient methods to identify the genetic variants governing them. Representation, distance and dispersion of splicing ratios We introduce a method to identify genetic variants associated with AS (sQTLs) in RNA sequencing population studies. In our approach, we define the splicing phenotype of a gene, as the distribution of the relative abundances of the gene’s alternative transcript isoforms. We use a distance-based approach to compute the variability of this multivariate phenotype across observations and a non-parametric analogue to MANOVA to compare this variability within and between genotypes. In what follows, we describe our approach in detail. The distribution of the abundances of individual transcript isoforms is the more general characterization of the splicing pattern of a gene since any other characteristic feature—exon or splice junction abundances or inclusions—can be derived from this distribution ( Fig. 1 ). To control for the effect of overall gene expression, we compute the relative abundance of the splicing isoforms to the total gene expression. For a specific gene, the relative abundance of the transcript i in observation j is , where x ij is the expression of isoform i in observation j and n is the number of isoforms of the gene. We will refer here to the relative transcript abundances f 1 j ,···, f nj for a gene, as the gene splicing ratios. Obviously, for any observation j . Geometrically, a gene with n transcript isoforms can be represented in a n -dimensional space, [0, 1] n , where the coordinates are the splicing ratios. Each point in this space defines a particular set of splicing ratios, different points corresponding to different observations. Because for any observation the sum of the splicing ratios is equal to one, the points are actually all located in the ( n −1) standard simplex subspace. The simplex generalizes the notion of the triangle in for instance, a 2-simplex is a triangle, a 3-simplex is a tetrahedron. An example for a gene with three isoforms is shown in Fig. 1 . Observations lying proximal in this space have similar splicing ratios. Different measures can be used in this space to define the distance between two observations. Here we have adopted the Hellinger distance that we proposed in Gonzalez-Porta [12] , which defines also the underlying metric of our approach. If f ij is the splicing ratio for isoform i of observation j , the Hellinger distance between j and k is: where n is the total number of isoforms in the investigated gene. The Hellinger distance is commonly used to measure the similarity of two probability distributions. For instance, the probabilities defining a multinomial distribution can also be represented by points in the simplex space and compared using this distance. The Hellinger distance has an interesting property for splicing ratios: compared with the Euclidean distance, it tends to exacerbate the differences between points near the edges of the simplex. In our case, those points at the boundaries of the space will have one major isoform expressed, with a high splicing ratio. As it has been previously reported [32] , we have also observed that for a substantial proportion of studied genes, a major isoform tend to capture most of the transcriptional output of the gene. The variability (or dispersion) within a set of N observations can be defined with the aid of the concept of centroid. For the Euclidean distance, the centroid is the average of all the points (observations). For non-euclidean distances (such as Hellinger distance) the centroid c is defined as the point that minimizes the sum of squared distances between itself and each point in the set of sampled points. As it will be detailed in the next section, the sum of squared distances ( SS ) between the N observations and the centroid is the basic measure of variability used in our approach: where is the squared Hellinger distance between the centroid c and observation j . In genes with similar splicing ratios across the individuals in the population, the dispersion of the points around the centroid is minimal and SS tends to 0. As the differences in AS ratios between individuals increase, SS increases, but is bounded by N −1 because the square of the Hellinger distance between two points in the ( n −1)-standard simplex is itself bounded by 2. Multivariate comparison of splicing ratios The Hellinger distance in the simplex allows to estimate and compare the variability of splicing ratios of a gene between and within groups of observations (genotypes in our case) using the test for location comparison introduced by Anderson [10] , [11] . This test is similar to a MANOVA without assuming any probabilistic distribution for the splicing ratios. It follows an analogous decomposition of the classic ANOVA, where the total variability SS T is partitioned in two complementary components, the within-group variability SS W and the between-group variability SS B : The Anderson test computes a pseudo-F ratio score that measures the relative difference between SS W and SS B . In the Anderson approach, the within (or residual) variability SS W is defined by the sum of the squared distances from individual observations to their group centroid ( Supplementary Fig. 2 ). The between-group sum of squares SS B is the sum of squared distances from the different group centroids to the overall centroid and the total variability SS T is defined by the sum of the squared distances from individual observations to the overall centroid. Anderson shows that the sum of squared distance between the samples to the centroid can be computed easily, without computing explicitly the centroid. Indeed, the sum of squared distances between points and their centroid is equal to the sum of squared interpoint distances divided by the number of points. Following Anderson notation, if N is the total number of observations: where is the Hellinger distance between the individuals j and k . The within-group variability is where p is the number of groups, n g the sample size of group g and ε g , j , k =1 if individuals j and k are sampled from group g , otherwise ε g , j , k =0. SS W is the weighted mean of the sum of squared interdistances within each group. Finally, The main advantage of this method is that it allows the usage of non-euclidean distances. Typically, permutations are performed to assess the significance of the F-scores. Because of their important computational cost, particularly in large data sets, we implemented an alternative approach using an approximation for the null distribution of the F-score. Following Anderson [14] , the null distribution is simulated through a ratio of two linear combinations of independent χ 2 variables with different degrees of freedom in the numerator and denominator. The coefficients of the linear combinations, both in the denominator and the numerator, are the eigenvalues of a matrix related to the interdistances’ matrix (see Anderson [14] for further details). Thanks to this approximation, the computation time of the multivariate test is not linearly dependent on the number of permutations anymore ( Supplementary Fig. 3a ). While the use of the approximation instead of permutations sped up the total sQTL analysis by a factor 3, the gain on the actual multivariate test is about 80-fold. We found that the results using this approximation were nearly identical to those obtained directly with permutations ( Supplementary Fig. 3b ). An important consideration concerns the homogeneity of the compared variabilities. As Anderson noticed, the location test is sensitive to group heterogeneity in the dispersion of points. Large heterogeneities may lead to significant differences for similar locations, that is, in the presence of different group dispersions, the location test may easily report a false significance. To test for the homogeneity of dispersions between two or more groups, we use a test also derived by Anderson [11] that adopts the same multivariate geometrical framework as the location test. The P values are obtained here with a permutation test. They allow us to identify and flag the cases where the dispersion of the compared groups is too large. Consequently, these flagged cases are not present in the results shown here. We used the betadisper method included in the vegan R package [33] to compute this score and the associated permutations. Parametric versus non-parametric approach Because of the nature of the data splicing ratios that configure multivariate simplex vectors, a non-parametric approach seems clearly preferable over a parametric one. Nonetheless, we have explored the possibility of using a MANOVA that requires multivariate normality of the data. To investigate whether MANOVA would be a good fit to our data, we have studied the distribution of two statistics commonly used in MANOVA analysis: Wilks’ lambda (Λ Wilks ) and Pillai's trace (Λ Pillai ). To compute the theoretical null distributions, we generated multivariate normal distributed values using the mean splicing ratios and their covariance matrix estimated from real data (CEU population in Geuvadis project). We simulated 90 samples (3 groups of 30 samples) and genes expressing 3, 4 and 7 isoforms. For each number of isoforms, we simulated 10,000 genes, computing and storing the Λ Wilks and Λ Pillai . On the other hand, for each gene expressing 3, 4 or 7 isoforms and SNP tested in the CEU population, we computed Λ Wilks and Λ Pillai on the real splicing ratios after shuffling the genotype groups to remove any true association. In that way, we derived good approximations of the real null distribution of both statistics, which can be compared with their null distributions under the multivariate normality assumption. As it is possible to see in Supplementary Fig. 4 , the distributions of both Λ Wilks and Λ Pillai simulated according to a multivariate normal distribution that depart substantially from the distributions obtained from the real data. This strongly suggests that the parametric approach is not an appropriate option to deal with our splicing ratios. We have already showed that we can use a very good asymptotic approximation to the null distribution ( Supplementary Fig. 3b ). Implementation of the sQTL discovery process We incorporated this method and representation into a QTL pipeline, and implemented the sQTLseekeR package. The pipeline takes as input a gene and transcript annotation on a given genome, and a collection of samples on which both, a set of SNPs and the expression levels of individual transcripts, have been determined. The pipeline identifies, first, the set of genes, samples and SNPs that are suitable for sQTLs analysis. Thus, we consider only genes with at least two splicing isoforms and genes exhibiting some minimal splicing variability across samples (specifically, for each gene we compute the mean distance to the centroid đ of the splicing ratios, Fig. 1 ) and, by default, consider only genes with >0.01. For each gene in this set, we consider only samples in which gene expression is over a given threshold (by default, ≥0.01 RPKM ). Similarly, for each gene, we consider only SNPs falling within the gene plus 5 kb upstream and downstream from the gene. The assumption here is that SNPs directly affecting the splicing pattern of a gene are likely to be carried out to the sequence of the primary transcript. From these SNPs, only bi-allelic SNPs creating at least two genotypic groups, each genotype present in at least five samples, are further considered. Then, for each gene–SNP pair, we group the samples according to their genotype and compute the F-score for the association between splicing ratios and genotype. As the Anderson's approach allows direct additive partitioning of variability for complex models, we used here a one-way factorial model with the genotype codes as levels of the factor. We prefer the factorial model to a regression model with the number of mutations as independent variable, because the factorial model is potentially able to detect more types of differences: additive, dominant, recessive or even undefined model changes. This is an advantage over the regression model because ratios could not follow strictly the additive model, as it is commonly accepted for changes in expression. Because the F-scores are sensitive to the heterogeneity of the variabilities between the genotype groups, we also perform a test of homogeneity of variabilities for each gene–SNP pair. Genes failing this test are flagged. Their significance is still assessed and they are taken into account to adjust the P values (see below), but they are not reported as significant sQTLs. To assess the significance of the F-score, we compute the null distribution at the gene level; that is, the same set of permuted/simulated values is used to assess the significance of all the SNPs tested for a gene. After all gene–SNP pairs are tested, the P values for all genes and all SNPs are pooled together and controlled for FDR using qvalue [31] R package with its default parameters. Details on the P value estimation We detail here some additional implementation details that improve the procedure to estimate P values. First SNPs creating only two genotypes have to be treated differently from those creating the three genotypes (reference/reference, reference/mutated, mutated/mutated) because the distribution of F-scores is sensitive to the number of groups compared. Thus, in practice, for each gene, we compute a different set of simulated/permuted scores for the SNPs creating two and three genotypes. Second, in Geuvadis computations, we are testing around 1.2 × 10 6 SNP–gene pairs per population ( Table 1 ). The FDR correction impels a priori to reach a higher number of different simulations/permutations per test. Fortunately, this large number is only needed for the highest scores, where maximum accuracy is critical. Thus, we attempt to use a number of computations tailored to each gene, avoiding useless computations. Intuitively, for high P values, just a few thousand values in the null distribution are sufficient to get usable accuracy for the downstream multiple-test correction. In practice, new simulated/permuted scores are computed until a minimum number (1,000 in Geuvadis analysis) of scores are found more extreme than the true score in the constructed null distribution, or the maximum number of simulations/permutations is reached. For Geuvadis analysis, we set this number to 3 × 10 6 . Finally, to ensure a robust F-score and an appropriate, that is, F-like, null distribution, an additional test verifies for each gene that at least 25 different splicing patterns are present in the total population and at least 5 different splicing patterns within every tested genotype group. Here a splicing pattern is the distribution of the splicing ratios for a gene. Indeed, if many samples have the exact same splicing ratios and, hence, fall in the exact same location, the F-score and its simulated (or even more its permuted) distribution might behave unreliably. This minimum number of truly different scores in the sample is not easy to establish because it is sensitive to the relative sizes of the genotype groups. We simulated a number of scenarios (where some individuals have different splicing configuration but the rest identical ones) where permutations are obtained taking the samples with replacement and performing a total of 2 × 10 6 tests. These simulations show a minimum required number of 25 different splicing patterns to obtain enough different configurations. Genes not satisfying these criteria are not tested. Workflow of Geuvadis sQTL discovery process Here we provide a detailed workflow of the sQTL discovery process that we have applied to the analysis of Geuvadis data set. First we identify genes suitable for the analysis, that is, genes with at least two alternative transcript isoforms and with splicing variability >0.01. Out of the 20,110 protein coding genes annotated in Gencode v12 (ref. 34 ), 16,581 have at least two annotated isoforms. Overall, 11,079 of these genes, on average per population, satisfied the minimum splicing variability criterion. Then for each suitable gene, we identify suitable samples and SNPs. Samples in which the expression of the gene is ≥0.01 RPKM are kept. Genes with less than 25 different splicing patterns in the population of surviving samples are further discarded. After this filter, 10,012 genes remained on average per population. Given a gene, SNPs where kept for subsequent analysis if located within a gene (or within 5 Kb upstream or downstream from the gene) and the two different alleles are present in the population. From the 10,785,347 SNPs originally in Geuvadis, on average 2,274,124 remained per population, after these two filters. These SNPs partition the population in two or three genotype groups. Furthermore, SNPs with less than five different splicing patterns in any of the genotype groups are further discarded. On average, 1,393,042 SNPs remained per population after this filter. For each suitable SNPs, we compute the F-score and save it in a list, separately for SNPs with two or three genotypes. Then for each list, the highest F-score is used to estimate the number of simulations/permutations needed to generate the null distribution. Finally, the simulated/permuted distribution is used to compute P values for the SNPs. After all genes have been tested, the P values are pooled and corrected using the qvalue R package for FDR control. For each suitable gene, we repeat the analysis described in the previous paragraph but now testing for homogeneity of variabilities across genotypes. After all genes have been tested again, the resulting P values are pooled and corrected. Significant sQTLs, surviving the homogeneity of variabilities test, are reported. Data and filters The Geuvadis project [8] produced RNA-Seq experiments for 465 samples from lymphoblastoid cell lines. A majority of these samples (422) were sequenced in the 1000 Genome Project Phase 1. The genetic variation from the other samples was imputed. RNA-Seq data were subjected to rigorous quality controls [35] . We used the transcript quantifications produced by Geuvadis in Gencode v12 (ref. 34 ). This data can be visualized or downloaded at www.ebi.ac.uk/Tools/geuvadis-das . Sharing of sQTLs across populations We compared the significance of the sQTLs across populations. Following the idea from Nica et al. [15] , we estimated the proportion of true association π 1 among the sQTLs from a first population in a second population. We also used qvalue R package to estimate π 1 as 1− π 0 . Estimation of the major AS event To characterize what type of AS events are preferentially affected by sQTLs, we employed the following strategy: given a sQTL, we identify the two transcript isoforms in the target gene that change the most between genotypes and exhibit symmetric behavior (example Fig. 2 , transcripts T1 and T2 ). Then, we compare the exonic structure of the two transcripts using the AStalavista [16] software. AStalavista provides an exhaustive characterization of all AS events when comparing the structure of all transcripts from a given locus. The comparison of two transcripts can sometimes be characterized by several distinct events affecting distinct regions of the transcript. Hence each sQTL can be associated to several events. Eventually, we can classify sQTL as affecting splicing of internal exons if at least one of the associated events involve internal exons. Here we have considered exon skipping, alternative 3′ and 5′ splice sites, intron retention, mutually exclusive exons, alternative 3′ and 5′ UTR, alternative first and last exon and tandem 3′ and 5′ UTR. These events are illustrated in Supplementary Fig. 5 . We grouped all other events in complex events categories: complex 3′/5′ event if changes only affected 5′/3′ termini without explicit splicing; complex splicing event when the splicing event could not be characterized by our nomenclature. As a control to assess enrichment of particular AS events, we randomly selected two transcripts from the genes associated to sQTLs and compared them using the same approach. Test on random gene–SNP pairing SNPs in a particular gene were tested for association with the splicing ratios of a different gene, selected randomly among the set of genes originally tested. In practice, the gene labels on the splicing ratios were simply shuffled. This test preserves the SNP correlation structure as all SNPs within a same gene will be tested against the splicing ratios of the same randomly selected gene. Functional analysis was then performed on the gene hosting the significant SNPs using DAVID [36] . Enrichment of sQTLs for biologically relevant features To assess the relevance of sQTLs, we tested the enrichment of a number of features, which are relevant from the biological standpoint. We tested for enrichment pooling sQTLs found in the five populations and compared the set of sQTLs (at FDR≤5%) against a set of non-sQTL SNPs (FDR>5%) with matched minor allele frequency. We assessed the significance of the enrichment using a Fisher test. We specifically tested for sQTLs falling more than expected in exons, splice sites, GWAS hits [37] or their vicinity (within 1 kb). We also compared the distance with the closest exon for intronic sQTLs and a set of intronic non-sQTLs with matched minor allele frequency. We used the Mann–Whitney test with the alternative hypothesis being intronic sQTLs are closer to exons than intronic non-sQTLs. Disruption of splice sites We investigated the extent of the splice site strength disruption by sQTLs compared with non-sQTLs. We used the absolute difference in the strength of the splice site between the reference allele sequence and the alternative allele sequence, Δscores. To compute the strength of donor and acceptor splice sites, we used standard position weight matrices [38] . To assess the significance of the difference between sQTLs and non-sQTLs, we the used Mann–Whitney test with the alternative hypothesis Δscores is higher for sQTLs than non-sQTLs. We expect that SNPs in splice sites increasing (decreasing) the splice site strength also increase (decrease) the usage of the splice site (as measured by RNA-Seq). We also expect this effect to be much stronger for SNPs that are sQTLs than for non-sQTL SNPs. We have therefore computed the enrichment of consistent changes (strength and usage of the splice site are positively correlated) over inconsistent changes (strength and usage of splice sites are negatively correlated) for both sQTL and non-sQTL SNPs occurring in splice sites. To compute the usage of a given splice site, we summed the relative abundance of the transcripts using the site. We then counted how many times an increase (or decrease) in the site strength coincides with an increase (or decrease) of its usage. We regressed the transcript relative abundance across the three genotype groups and required a minimum regression slope (minimum 5% change in the site usage from one genotype group to another) along with a minimum strength score change (0.1) in the relevant direction to declare the changes consistent. Splice sites used by all or none of the expressed transcripts were not included here because they could not show any usage variation. We then computed the ratio of consistent over inconsistent changes for both sQTL and non-sQTL SNPs occurring in splice sites. We expect almost no enrichment for non-sQTLs and a larger enrichment for sQTLs. Overlap with previous studies Kwan et al. [17] used exon array to detected sQTLs in Hapmap samples. Twenty-five sQTLs were experimentally validated. Although on the same population (CEU), the samples used in Geuvadis were not exactly the same. The technology is also different for both expression and genotypes information: RNA-Seq versus exon array and sequencing versus SNP-array, respectively. Simulation of the univariate and multivariate approaches We have used simulations to further compare the univariate and multivariate approaches. We have considered genes with 3, 4, 7, 10 and 15 isoforms—numbers that capture the wide spectrum of splicing complexity of human genes ( Supplementary Figure 5 ). We estimated the mean splicing ratios and the covariance matrix from real data (CEU population in Geuvadis project). Genes were compared in two simulated populations of 40 individuals each. To create differences in the splicing ratios, the mean values of the transcript isoforms with relative abundance were shifted in one population with respect to the other. This shift captures the effect size of the differences in splicing ratios between the two populations: a stronger shift (effect) will create clearer differences, hence easier to detect (see below). Moreover, the shift in average splicing ratios in the second population can be distributed differently across the transcript isoforms. While each gene is likely to have its characteristic splicing pattern, we have chosen to simulate four basic scenarios, which we believe capture a broad spectrum of biological cases. In the first scenario, labeled ‘first and second major transcripts only’, only the splicing ratios of the first two major transcripts, that is, most expressed, are shifted in the second population. In the second scenario, ‘second and third major transcripts only’, only the splicing ratios of the second and third major isoforms are changed in the second population. In the third scenario, ‘all transcripts’, the splicing ratios of all transcript are shifted with the same intensity in the second population. Finally, the splicing ratios of all transcripts are shifted but the value of the change in the major isoform is distributed equally among the rest of the isoforms, that is, the major transcript changes strongly while the other transcripts change slightly (‘first transcript strong, others weak’). For each scenario, we simulated 20 effect sizes of varying magnitude. In total, therefore, we simulated 400 different configurations. For each configuration, 5,000 genes were simulated: 500 with shifted average splicing ratios as explained before and 4,500 with similar distribution in both groups. This design was chosen to mimic a genome-wide analysis. Then the P values from univariate and multivariate approaches were corrected for multiple testing using the Benjamini–Hochberg algorithm and the true positive rate at FDR 1% is reported. Results are shown in Fig. 6 . The multivariate approach consistently detects more significant associations in almost all configurations, than the univariate approach. For some effect sizes, the univariate approach misses almost half of the associations identified by the multivariate approach. To explore how realistic are the effect sizes in which the multivariate approach outperforms the univariate approach, we estimated effect sizes on Geuvadis data using real and simulated SNPs. That is, we computed the distribution of effect sizes in partitions of the CEU population induced by real SNPs, and generated randomly. We expect some of the partitions induced by real SNPs to be associated with changes in the splicing ratios, but not the random partitions. To measure the effect size consistently with the simulations (the distributed shift on the average splicing ratios), we sum the absolute differences in average splicing ratios between the two groups divided by two. The distributions of effect sizes are plotted in Supplementary Fig. 1 . There is a shift towards higher effect sizes in real compared with random partitions. It is at this larger effect sizes (from 0.1 to 0.25, see Fig. 6 ) that the multivariate approach outperforms the univariate approach, suggesting that the former is able to detect biologically relevant associations that escape the univariate approach. Transcript QTLs Transcript QTLs (trQTLs) were identified using Geuvadis eQTL pipeline [8] on transcript ratios. SNPs located closer than 1 Mbp to the gene TSS were tested for association with each transcript independently. The four European populations were pooled together to increase the discovery power. The results can be downloaded from http://www.ebi.ac.uk/Tools/geuvadis-das/ . Summary table and methodological details can be found in Geuvadis article [8] . Enrichment and splice site disruption analysis were performed similarly than for sQTLseekeR sQTLs. Exon centric sQTLs Exon inclusion levels were estimated from the RNA-Seq reads produced by the Geuvadis consortium. For each internal exon (with at least an upstream and downstream exon) from genes with three or more exons, we computed the so-called percentage splice index (PSI). We computed this index as previously proposed [39] , [40] . The index is computed from three values: (A) the number of reads that map in the exon body, (B) the number of split reads mapping to splice junctions between the considered exon and both adjacent exons and (C) the number of split reads mapping to the splice junction from the adjacent exon upstream to the adjacent exon downstream. A and B represent reads that support exon inclusion and C reads that support exon exclusion. Then, PSI is computed as PSI=A+B/(A+B+C). PSI=0 means that the tested exon is not included, whereas PSI=1 indicates that the exon is constitutively spliced in. Since the majority of the exons have low variability, we selected only those exons with a PSI coefficient of variation >0.05 per population and with missing values in less than 10% of the population samples. Missing PSI values were imputed using the median PSI value for the exon across the population. We used Spearman rank correlation to test for association between PSI levels and genotype. We limited the variants tested to those present in a 5 KB window surrounding the middle of the exon. We assess significance by computing the FDR using the qvalue package [31] . We reported significant associations (psiQTLs) at 1% FDR. Because this approach dealt with a different splicing metric, filtering steps lead to different set of gene–SNP being tested ( Table 3 ). Focusing on the gene–SNP tested in both approaches enrichment and splice site disruption analysis were performed as described previously (Section enrichment of sQTLs for biologically relevant features, Table 4 , Fig. 5 ). How to cite this article : Monlong, J. et al. Identification of genetic variants associated with alternative splicing using sQTLseekeR. Nat. Commun. 5:4698 doi: 10.1038/ncomms5698 (2014).